Visualizing influenza virus infection in living mice Preventing and treating influenza virus infection remain a challenge because of incomplete understanding of the host–pathogen interactions, limited therapeutics and lack of a universal vaccine. So far, methods for monitoring the course of infection with influenza virus in real time in living animals are lacking. Here we report the visualization of influenza viral infection in living mice using an engineered replication-competent influenza A virus carrying luciferase reporter gene. After intranasal inoculation, bioluminescence can be detected in the chest and nasopharyngeal passage of living mice. The intensity of bioluminescence in the chest correlates with the dosage of infection and the viral load in the lung. Bioluminescence in the chest of infected mice diminishes on antiviral treatment. This work provides a novel approach that enables real-time study of influenza virus infection and effects of antiviral therapeutics in living animals. Influenza viruses cause seasonal epidemics and occasional threats as seen with ‘swine’influenza H1N1, avian influenza H5N1 and very recently H7N9 viruses in humans that resulted in significant morbidity and mortality [1] . A better understanding of the viral infection and development of better therapeutics and vaccines would help to alleviate this burden. Animal models, especially mice, are commonly used in studying influenza virus. However, conventional studies in mice rely on monitoring survival, euthanizing animals and dissecting tissues at multiple time points to assess viral infection, host response and to evaluate the efficacy of vaccines and antiviral therapeutics. So far, there is no good method for real-time monitoring of influenza viral infection in living animals. Therefore, an influenza virus carrying a bioluminescence reporter should be of great value for studying this viral infection and for evaluating antiviral therapeutics and vaccines in living animals. The genome of influenza A virus (IAV) contains eight negative-sense, single-strand viral RNA (vRNA) segments. The mechanism utilized by IAV to assemble these eight vRNA segments into the virion is not fully understood. Several studies suggested that the packaging signals residing in both 3′- and 5′-non-coding regions and coding sequences at two ends of each open reading frame have critical roles in specifically packaging each segments into a complete virion [2] , [3] , [4] , [5] . Efforts have been made to insert exogenous genes into its genome, especially insertion of the gene-encoding green fluorescent protein (GFP) into the neuraminidase (NA) and haemagglutinin (HA) segments. However, such manipulations usually were achieved at the cost of replacement or truncation of the original open reading frames in these segments. Thus, the production of such recombinant IAVs requires either creating complementary cell lines that provide HA in trans [4] , [6] or in the case of NA deletion, adding exogenous NA protein to the culture medium [7] or developing specific cell lines that express low sialic acid [3] . The deletion or truncation of HA- or NA-coding sequence from the viral genome limits viral replication in non-complementary cells and prohibits large-scale production in embryonated chicken eggs. Deletion or truncation or fusion of key viral components critical for viral infection such as HA, NA or NS1 would usually devalue the usefulness of these genetically modified influenza viruses in animal model studies. Recently, we and another lab described the generation of a replication-competent IAV expressing GFP either through insertion of a GFP gene into the NA segment [8] or expressing a NS1–GFP fusion protein through NS segment engineering [9] . However, because of interference from high background fluorescence, these influenza viruses were not useful for real-time monitoring of influenza virus infection in living mice [9] . We report here the generation of a replication-competent IAV expressing Gaussia luciferase (IAV-Luc). Dose-dependent bioluminescence can be detected in the chest of living mice after intranasal inoculation with IAV-Luc, and the intensity of bioluminescence correlates with the viral load in the lungs and diminishes on treatment with an antiviral serum. This work provides a new approach for real-time study of influenza virus infection and evaluation of antiviral therapeutics in vivo and in vitro . Characterization of influenza virus expressing luciferase We first generated a replication-competent IAV that is capable of expressing bioluminescence protein luciferase (IAV-Luc). Using influenza A/Puerto Rico/8/34 (PR8) as the backbone, we constructed IAV-Luc by inserting the codon-humanized gene-encoding Gaussia luciferase into the C-terminal of the full-length NA-coding sequence linked by a 2A autoproteolytic cleavage sequence. Gaussia luciferase is the smallest luciferase in its family and has a short half-life of 20 min in vivo [10] , These features make it an ideal reporter for our purpose. We retained the 5′- and 3′-terminal regions of the chimeric NA segment containing 157 nucleotides and 183 nucleotides of the original non-coding and coding sequences in the NA segment, which have been shown to be required for efficient packaging of NA segment into the virion [2] , [3] ( Fig. 1a ). We then successfully rescued IAV-Luc by transfecting 293T cells using an eight-plasmid reverse genetics system and propagated in embryonated chicken eggs. 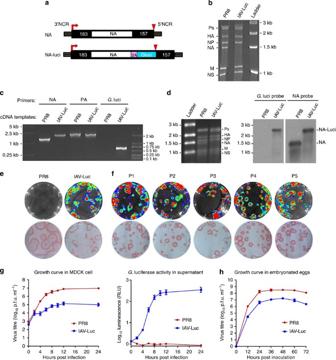Figure 1: Generation and characterization of replication-competent IAV carrying luciferase reporter (IAV-Luc). (a) Schematic representation of influenza NA vRNA segment in IAV-Luc. The gene-encodingGaussialuciferase was inserted into the C-terminal region of NA linked by a 2A autoproteolytic cleavage sequence. (b) PAGE analysis of RNA samples extracted from IAV-Luc and PR8 virions. (c) PCR using specific primers for PA, NA and luciferase to confirm the size of chimeric NA segment and the insertion of gene-encodingGaussialuciferase. (d) Analysis of RNA samples extracted from IAV-Luc and PR8 virions by agarose gel electrophoresis followed by northern blot using specific probes for NA andGaussialuciferase. (e) Plaques on MDCK monolayer cells formed by IAV-Luc showed bioluminescence on addition of luciferase substrate coelenterazine. The same culture dishes were immunostained using anti-NP antibodies to reveal all plaques. (f) Plaques on MDCK monolayer cells formed by IAV-Luc from passages one to five. (g) Growth kinetics of parental PR8 and IAV-Luc in MDCK cells infected with virus at MOI of 1. The viral titres (Log10p.f.u. ml−1) and luciferase activities (Log10relative light units (RLU)) were determined at indicated time points after infection. (h) Growth kinetics of parental PR8 and IAV-Luc in chicken-embryonated eggs. Each data point represents mean±s.e.m. (n=3). Figure 1: Generation and characterization of replication-competent IAV carrying luciferase reporter (IAV-Luc). ( a ) Schematic representation of influenza NA vRNA segment in IAV-Luc. The gene-encoding Gaussia luciferase was inserted into the C-terminal region of NA linked by a 2A autoproteolytic cleavage sequence. ( b ) PAGE analysis of RNA samples extracted from IAV-Luc and PR8 virions. ( c ) PCR using specific primers for PA, NA and luciferase to confirm the size of chimeric NA segment and the insertion of gene-encoding Gaussia luciferase. ( d ) Analysis of RNA samples extracted from IAV-Luc and PR8 virions by agarose gel electrophoresis followed by northern blot using specific probes for NA and Gaussia luciferase. ( e ) Plaques on MDCK monolayer cells formed by IAV-Luc showed bioluminescence on addition of luciferase substrate coelenterazine. The same culture dishes were immunostained using anti-NP antibodies to reveal all plaques. ( f ) Plaques on MDCK monolayer cells formed by IAV-Luc from passages one to five. ( g ) Growth kinetics of parental PR8 and IAV-Luc in MDCK cells infected with virus at MOI of 1. The viral titres (Log 10 p.f.u. ml −1 ) and luciferase activities (Log 10 relative light units (RLU)) were determined at indicated time points after infection. ( h ) Growth kinetics of parental PR8 and IAV-Luc in chicken-embryonated eggs. Each data point represents mean±s.e.m. ( n =3). Full size image We first confirmed that the chimeric NA segment was packaged into the virion by analysing purified vRNA on 3.5% of polyacrylamide gel electrophoresis (PAGE). As the chimeric NA vRNA segment of IAV-Luc has insertion of the gene-encoding Gaussia luciferase, its size increased from 1.4 to 2.2 kb, which falls into the range of polymerases gene fragments (PB1, PB2 and PA) on the RNA PAGE. The sizes and ratios of all other segments showed no visible changes ( Fig. 1b ). Both northern blot analysis and reverse transcriptase-PCR using specific primers for genes encoding NA and luciferase confirmed the integrity of the chimeric NA segment containing both NA and luciferase, as well as the packaging of the chimeric NA vRNA into the virion ( Fig. 1c,d ). We then confirmed that IAV-Luc expresses luciferase using the Xenogen IVIS200 imaging system. In parallel with immunochemical staining using an anti-influenza nucleoprotein (NP) antibody for the same culture plate, all plaques formed by IAV-Luc on Madin–Darby canine kidney (MDCK) monolayer cells were positive for bioluminescence on addition of the luciferase substrate coelenterazine ( Fig. 1e ). However, the plaques formed by IAV-Luc were somewhat smaller than the plaques formed by PR8 virus, indicating that IAV-Luc has a slower growth rate than the parental PR8 virus. To test whether the inserted gene and the chimeric NA segment could be stably maintained in the viral genome, we consecutively propagated IAV-Luc in 10-day-old embryonated chicken eggs for five passages. Plaques formed by IAV-Luc from passages one to five were all bioluminescence-positive as compared with the immunostaining using anti-NP antibody for the same plates ( Fig. 1f ). Sequencing analysis showed no mutations in the chimeric NA segment for IAV-Luc purified from passage one to five. We next compared the growth kinetics of IAV-Luc with the parental PR8 virus in MDCK cells and embryonated chicken eggs ( Fig. 1g,h ). Viral titres in the culture supernatant or allantoic fluid were quantified at various time points after infecting MDCK cells. In a single-cycle replication assay (multiplicity of infection (MOI)=1), the replication of IAV-Luc in 24 h was 1 × 10 5 p.f.u. ml −1 as compared with 9 × 10 6 p.f.u. ml −1 for parental PR8 virus. The activities of luciferase in supernatant could be detected as early as 2 h post infection and increased over time. In embryonated chicken eggs, the yield of IAV-Luc at 48 h post infection could reach up to 1.8 × 10 7 p.f.u. ml −1 of allantoic fluid compared with 3.2 × 10 8 p.f.u. ml −1 for the parental PR8 virus. This result demonstrated that the growth of IAV-Luc is robust enough for production in embryonated chicken eggs for practical research application. Bioluminescence imaging of IAV-Luc infection in living mice We assessed whether bioluminescence could be detected in the mice infected with 10 6 p.f.u. of IAV-Luc via intranasal inoculation. At 48 h post infection, we anaesthetized and observed live mice using the Xenogen IVIS200 imaging system after injection of the substrate coelenterazine. Bioluminescence could be observed in the chest of IAV-Luc-infected mice within 10 min after intravenous injection of coelenterazine but not in PR8-infected mice. Next, the lungs from IAV-Luc and PR8-infected mice were imaged after perfusion with a buffer containing coelenterazine. Again, only the lungs of the IAV-Luc mice were positive, confirming that the bioluminescence observed in the chest was the result of IAV-Luc infection in the lungs ( Fig. 2a ). Interestingly, we also detected a weaker bioluminescence signal in the nasopharyngeal passage of these mice because intranasal inoculation was used as the route to initiate the infection. We then assessed for dose dependency of bioluminescence with infection dosage. At 48 h post infection, photon flux in the chest and nasopharyngeal passage could be detected in mice that received 10 5 p.f.u. of IAV-Luc. The intensity of this photon flux in these regions significantly increased with 10 6 p.f.u. However, the elevation of bioluminescence intensities from 10 6 to 10 7 p.f.u. infection dosages was less drastic, possibly because of saturation of the infection via intranasal inoculation ( Fig. 2b,c ). Further, we monitored the duration of bioluminescence that could be detected in mice after infection with 10 6 p.f.u. IAV-Luc. Bioluminescence could be detected at 1 day after infection, peaked at 2 days and remained detectable for at least 6 days after initiating the infection ( Fig. 2d ). To determine whether there was a direct correlation between the bioluminescence intensity and the viral titre in the lung, we collected the lungs from mice at 2–6 days post infection to measure viral load by plaque formation assay. We observed a good correlation ( R 2 =0.92) between bioluminescence intensity and the viral load in the lungs, validating the use of bioluminescence as a marker to assess the viral load in the lungs of mice infected with IAV-Luc ( Fig. 2e,f ). Clearly, these results indicate that bioluminescence imaging in IAV-Luc-infected living mice can accurately reflect the status of pulmonary infection in real time. 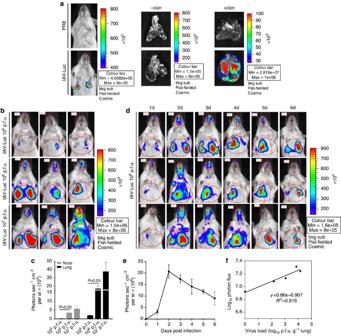Figure 2: Bioluminescence imaging of mice infected with LAV-Luc via intranasal inoculation. (a) Living mice infected with 106p.f.u. of IAV-Luc or 103p.f.u. of PR8 were imaged at 48 h post infection after injection of coelenterazine. The lungs were dissected and imaged after perfusion of coelenterazine. (b) Mice infected with 105, 106and 107p.f.u. of IAV-Luc were imaged at 48 h post infection after injection of coelenterazine. (c) Values of photon flux for each infection dosage group; each data point represents mean±s.e.m. (n=3). The statistical significance of differences was calculated using Student’st-test. (d) Mice infected with 106p.f.u. of IAV-Luc were imaged from 1 to 6 days post infection. (e) Values for photon flux from 1 to 6 days post infection; each data point represents mean±s.e.m. (n=3). (f) Correlation of viral load in the lungs to photon flux in the chests from day 2 to day 6 post infection. Each data point represents mean±s.e.m. (n=3) from mice infected with 106p.f.u. of IAV-Luc. Figure 2: Bioluminescence imaging of mice infected with LAV-Luc via intranasal inoculation. ( a ) Living mice infected with 10 6 p.f.u. of IAV-Luc or 10 3 p.f.u. of PR8 were imaged at 48 h post infection after injection of coelenterazine. The lungs were dissected and imaged after perfusion of coelenterazine. ( b ) Mice infected with 10 5 , 10 6 and 10 7 p.f.u. of IAV-Luc were imaged at 48 h post infection after injection of coelenterazine. ( c ) Values of photon flux for each infection dosage group; each data point represents mean±s.e.m. ( n =3). The statistical significance of differences was calculated using Student’s t -test. ( d ) Mice infected with 10 6 p.f.u. of IAV-Luc were imaged from 1 to 6 days post infection. ( e ) Values for photon flux from 1 to 6 days post infection; each data point represents mean±s.e.m. ( n =3). ( f ) Correlation of viral load in the lungs to photon flux in the chests from day 2 to day 6 post infection. Each data point represents mean±s.e.m. ( n =3) from mice infected with 10 6 p.f.u. of IAV-Luc. Full size image IAV-Luc could cause pathogenicity in mice The PR8 virus is a highly adapted influenza virus strain in mice that could cause disease symptoms and mortality in mice. To test whether IAV-Luc could confer pathogenicity in mice, we infected BALB/c mice with IAV-Luc via intranasal inoculation. Mice infected with 10 3 , 10 4 , 10 5 and 10 6 p.f.u. had dose-dependent loss of body weight and lethality ( Fig. 3a ). Mice infected with 10 6 p.f.u. IAV-Luc had similar weight loss and lethality as infection with 10 3 p.f.u. of PR8. All mice in these two groups were euthanized by day 6–7 after infection and histopathological examination showed that the lungs collected from mice at 5 days after infection with IAV-Luc had alveolar damage and interstitial inflammatory infiltration ( Fig. 3b ). These results demonstrated that IAV-Luc could confer pathogenicity in mice and thus could be exploited for real-time monitoring of infection status and for evaluation of antiviral therapeutics. 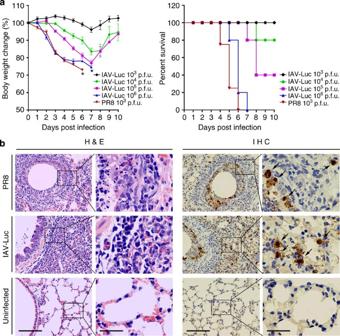Figure 3: Infection of IAV-Luc in mice resulted in loss of body weight and lung injuries as well as lethality. (a) Mice infected with either 103, 104, 105, 106p.f.u. of IAV-Luc or 103p.f.u. of PR8 were monitored daily for body weight and survival (mean±s.e.m.,n=5), * indicates the day all mice died of infection. (b) Histopathological analysis of lungs at day 5 after infection with 106p.f.u. of IAV-Luc or 103p.f.u. of PR8. Tissue sections of lungs were stained with haematoxylin and eosin or by immunohistochemistry using a mouse anti-NP mAb. Scale bar, 100 μm in the first and third columns and 25 μm in the second and fourth columns. Figure 3: Infection of IAV-Luc in mice resulted in loss of body weight and lung injuries as well as lethality. ( a ) Mice infected with either 10 3 , 10 4 , 10 5 , 10 6 p.f.u. of IAV-Luc or 10 3 p.f.u. of PR8 were monitored daily for body weight and survival (mean±s.e.m., n =5), * indicates the day all mice died of infection. ( b ) Histopathological analysis of lungs at day 5 after infection with 10 6 p.f.u. of IAV-Luc or 10 3 p.f.u. of PR8. Tissue sections of lungs were stained with haematoxylin and eosin or by immunohistochemistry using a mouse anti-NP mAb. Scale bar, 100 μm in the first and third columns and 25 μm in the second and fourth columns. Full size image Real-time imaging of antiviral agent in vitro and in vivo We next tested whether IAV-Luc can be used for evaluating antiviral therapeutics. As a proof-of-principle, we used an antiviral serum collected from convalescent mice previously infected with PR8 to test whether IAV-Luc could be applicable for evaluating antiviral therapeutics. We first incubated IAV-Luc with serial dilutions of the antiviral serum and then infected MDCK cells in 96-well plates. At 24 h post infection, we determined the bioluminescence intensity. As reflected by the value of photon flux, IAV-Luc could be completely inhibited by antiviral sera with 1:500 dilution at MOI of 0.5 or with 1:2500 dilution at MOI of 0.05 ( Fig. 4a ). These results demonstrated the potential of using IAV-Luc for developing viral neutralization assays for in vitro evaluation of antiviral drugs. 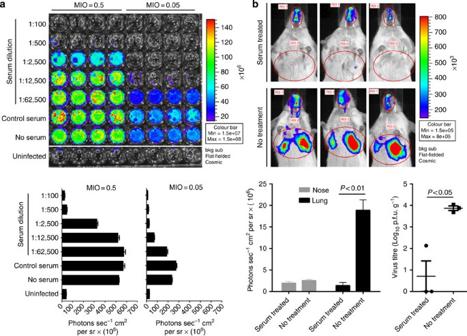Figure 4: Bioluminescence imaging of IAV-Luc could be exploited to evaluate antiviral therapeuticsin vitroand in living mice. (a) Dilutions of IAV-Luc were incubated with serial dilutions of the antiviral serum and then added to MDCK cells cultured in 96-well plates. Bioluminescence was measured at 24 h post infection. Complete neutralization of IAV-Luc resulted in no detection of luciferase activity. Each data point represents mean±s.e.m. (n=4). (b) Bioluminescence imaging of mice and analysis of photon flux at 48 h post infection. Mice infected with 106p.f.u. of IAV-Luc were untreated or treated with 100 μl of antiviral serum. The Lung viral load was determined after the bioluminescence imaging. Each data point represents mean±s.e.m. (n=3). The statistical significance of differences were calculated using Student’st-test. Figure 4: Bioluminescence imaging of IAV-Luc could be exploited to evaluate antiviral therapeutics in vitro and in living mice. ( a ) Dilutions of IAV-Luc were incubated with serial dilutions of the antiviral serum and then added to MDCK cells cultured in 96-well plates. Bioluminescence was measured at 24 h post infection. Complete neutralization of IAV-Luc resulted in no detection of luciferase activity. Each data point represents mean±s.e.m. ( n =4). ( b ) Bioluminescence imaging of mice and analysis of photon flux at 48 h post infection. Mice infected with 10 6 p.f.u. of IAV-Luc were untreated or treated with 100 μl of antiviral serum. The Lung viral load was determined after the bioluminescence imaging. Each data point represents mean±s.e.m. ( n =3). The statistical significance of differences were calculated using Student’s t -test. Full size image To address the possibility of using IAV-Luc for assessment of antiviral therapeutics in living mice, we first infected mice with 10 6 p.f.u. of IAV-Luc via intranasal inoculation and then treated with 100 μl of antiviral serum at 1 h after infection. At 48 h post infection, mice treated with antiviral serum treatment had no or little bioluminescence in the chests, whereas the mice who received no antiviral serum displayed strong bioluminescence signals ( Fig. 4b ). It is important to note that monitoring the change of body weight and survival at 48 h post infection were not able to depict any significant differences between treated and untreated groups. We also determined the viral load in the same lungs by dissecting and homogenizing the lung tissues for plaque formation assay. The viral load in serum-treated lungs was over 4-logs lower than that in the untreated group. This result confirmed that bioluminescence image analysis of IAV-Luc-infected mice can predict the therapeutic outcome. It is also interesting to note that the decrease of bioluminescence in the nasopharyngeal region of treated mice was not as dramatic as that in the chest. This may be because of possibly poor distribution of antiviral antibodies to the nasopharyngeal passage, as intravenously administered antiviral serum lack of dimeric or secretory IgA that contributes to protect the nasopharyngeal mucosa from viral infection. This observation suggests that the clearance of virus in the nasopharyngeal passage may lag behind that in the lung in the case of antiviral therapies using antiviral serum or IgG based antibodies. Our work provided a unique approach for studying influenza virus infection and evaluating antiviral therapeutics in living animals in real time. Although several other viruses such as herpes simplex virus, sindbis virus, vaccinia virus and dengue virus expressing luciferase for bioluminescence imaging in living mice have been reported [11] , [12] , [13] , [14] , our study was among the firsts to successfully demonstrate a replication-competent IAV that can express luciferase on infection in cultured cells or in mice. Importantly, our vector enables bioluminescence imaging of infection status without killing the mice. The development of such a virus will allow the status of viral infection in living animals to be monitored in real time and the infection progression to be followed longitudinally over time for the same animal. The number of animals needed to collect sufficient data could potentially be reduced. Using IAV-Luc for bioluminescence imaging analysis of viral infection, the efficacy of antiviral therapeutics could be detected earlier before the change of body weight or survival. In our proof-of-principle experiment to evaluate antiviral therapeutics in living mice, we observed a significant reduction in bioluminescence signal in mice who received antiviral serum at 48 h post treatment, which correlated well with the lung viral load. In contrast, it usually takes more days to observe the antiviral effect reflected by the difference in body weight and survival in infected mice. We note that IAV-Luc may also provide new insights in developing antiviral therapeutics. On treatment with antiviral serum, the reduction of bioluminescence in the nasopharyngeal passage lags behind that in the lungs, indicating the possibility that intravenous administration of serum- or IgG-based therapeutics may not be able to clean the IAV in the nasopharyngeal passage as fast as the lung. We propose that although the antiviral IgG in the serum can be distributed readily through the systemic circulation, dimeric IgA or secretory IgA, which is scarce in the serum, thus may not be presented to the nasopharyngeal mucosa site to exert protection. This suggests that a nasal spray for antibody delivery or other inhalation-based modalities to the nasopharyngeal passage may need to be applied to clean the virus in the nasopharyngeal passage for minimizing transmission. During the revision of this paper, an independent work by Heaton et al. [15] was published, in which the Gaussia luciferase gene was inserted into a different vRNA segment, PB2. In this paper, the virus was used to characterize monoclonal antibodies (mAbs) that bind to the conserved stalk domain of the viral HA of H1 and H5 subtypes, although the analysis was performed by measuring luciferase activities in lung homogenates but not in living animals. The insertion of luciferase gene into different vRNA segments may provide more options to apply these bioluminescence viruses for different research usages. It would be interesting if these two viral constructs could be compared in future experiments. Although Gaussia luciferase was used as it is the smallest luciferase gene identified so far that enable us to successfully engineer a replication-competent IAV, its blue light emission peaks at 490 nm wavelength which could be absorbed by tissue chromophores such as haemoglobin and thus lead to the loss of sensitivity. Further, the pharmacokinetics and bioavailability of the substrate coelenterazine is not ideal; it requires the imaging of animals to be performed immediately after the injection of ethanol-dissolved coelenterazine. Recently, a water-soluble coelenterazine was reported that could yield up to 100-fold greater sensitivity compared with native coelenterazine for in vivo imaging [16] . Therefore, future studies using this new substrate may provide better information output and sensitivity that can further facilitate the use of this technology for real-time analysis of viral infection. Although the primary objective of this work was to demonstrate real-time visualizing IAV infection in living animals, it could also be exploited for developing in vitro assays for screening antiviral drugs. Future studies will be needed to further explore the use of such visible IAV in studying viral biology, pathogenesis and developing new therapeutics. Cells and key reagents Human embryonic kidney 293T cells and MDCK cells were maintained in DMEM (Invitrogen) supplemented with 10% heat-inactivated fetal bovine serum (Hyclone) and antibiotics (100 μg penicillin ml −1 and 100 μg streptomycin ml −1 ). The antibody to influenza NP was purchased from Southern Biotechnology (Alabama, USA). Construction of IAV expressing luciferase A plasmid named pM-PR8-NA-2A-Gluc for expressing NA segment was constructed by inserting gene-encoding Gaussia luciferase into the C-terminal of NA gene inframely linked by the 2A autocleavage peptide sequence GSGATNFSLLKQAGDVEENPGP [17] . Viruses were rescued as described previously [8] , [18] . Briefly, 1 μg of the plasmid pM-PR8-NA-2A-Gluc, together with 1 μg each of other seven PR8 pM plasmids were combined with 16 μl of transfection reagent Lipofectamine 2000 (Invitrogen) for transfection of 293T cells. Forty-eight hours after transfection, culture medium was collected and subsequently inoculated into the allantoic cavities of 10-day-old embryonated chicken eggs for virus propagation. Propagation and purification of IAV At 48 h after ioculating virus into the allantoic cavities of 10-day-old embryonated chicken eggs, allantoic fluids containing influenza virus were collected and clarified by centrifugation at 6,000 r.p.m. at 4 °C for 15 min using a Beckman rotor SW28. Clarified supernatant was then layered onto a 30% sucrose cushion and further centrifuged at 25,000 r.p.m. for 2.5 h. Purified viruses were suspended in PBS buffer supplemented with 0.5% of BSA and stored at −80 °C. PAGE analysis of vRNA vRNAs were extracted from the purified viruses using MagMAX Viral RNA Isolation Kit (Ambion). vRNA samples were electrophoresed in a 3.5% polyacrylamide gel containing 7 M urea at 80 V for 5 h. RNA molecules were visualized using SYBR Green II RNA Gel Stain (Invitrogen) according to the manufacturer’s protocol. Reverse transcriptase-PCR analysis of vRNA VRNA of IAV-Luc and PR8 were extracted from allantoic fluid with the RNeasy Mini Kit (Qiagen). Complementary DNA was prepared using reverse transcriptase (SuperScript III; Invitrogen) and 5′-phosphorylated uni-12 primer (5′-AGCA/GAAAGCAGG-3′), which is based on the consensus 3′-sequence of the vRNA end sequences of the IAV. Primer pairs complementary to the NA and PA gene segments, the Gaussia luciferase primer pairs complementary to the NA and PA gene segments and the Gaussia luciferase are as follows: NA (5′-AGCGAAAGCAGGGGTTTAAAAT-3′, 5′-AGTAGAAACAAGGAGTTTTTTGA A-3′); PA (5′-AGCGAAAGCAGGTACTGATC-3′, 5′-AGTAGAAACAAGGTACTTTTTTGG-3′); Gluci (5′-ATGGTGAATGGCGTGAAG-3′, 5′-TAGGTGTCATCGCCGCCAGC-3′). Northern blot analysis of vRNA Five hundred nanograms of total RNA extracted from purified viruses were separated by 1% formaldehyde denaturing agarose gel electrophoresis and then transferred to a positively charged nylon membrane (Ambion) by pressure blotter method. Single-stranded biotin-labelled RNA probes were prepared using a MAXIscript SP6 Kit (Ambion). Target sequences (about 400 bp) were amplified by PCR using NA or Gaussia luciferase DNA as a template and then cloned into the pGEM-4Z vector (Promega) at the 3′-termini of SP6 promoter. Primer pairs for NA and Gaussia luciferase target sequences are as follows: NA (5′-CCGGAATTCTCGGTTGCTTGGTCAGCAAG-3′, 5′-CCCAAGCTTTTTGATCGAAAGACACCC AT-3′); Gaussia luciferase (5′-CCGGAATTCATGGTGAATGGCGTGAAGGT-3′, 5′-CCCAAGCTTCAATGAAC TGCTCCATGGGC-3′). The resulted plasmid DNA were linearized and then used as a DNA template for an in vitro transcription reaction using the MAXIscript SP6 Kit and biotin-16-UTP (Ambion). Hybridization was carried out in ULTRAhyb medium (Ambion) overnight at 68 °C. Blots were washed using NorthMax Low Stringency Buffer and with NorthMax High Stringency Buffer (Ambion). Northern blots were developed using alkaline phosphatase and streptavidin according to manufacturer’s protocols (BrightStar BioDetect; Ambion). Analysis of viral growth in cells and chicken eggs Growth curves were used to analyse the replication characteristics of IAV-luc virus. Confluent monolayers of MDCK cell in 35 mm dish were inoculated with diluted virus at a MOI of 1. After incubation for 1 h at 37 °C, the virus suspension was removed and replaced with 3 ml of DMEM containing 0.3% BSA (Invitrogen) and 1 μg ml −1 trypsin, N-tosyl- L -phenylalanyl chloromethyl ketone (TPCK) treated (Sigma-Aldrich). At given time points, 200 μl of culture supernatant was collected for virus titration and was replenished with same amount of fresh medium. The luminescence activities of the culture samples were also detected with luciferase assay reagent (Progema) as per the manufacture’s instruction. The viral titres at each time point were determined by plaque formation assay. Ten-day-old embryonated chicken eggs were inoculated with 100 EID 50 of virus. Allantoic fluid was collected at 12-h intervals. The viral titres at each time point were determined by plaque formation assay. Plaque formation assay Confluent MDCK cell monolayers in 12-well plates were infected with 10-fold dilutions of virus in a total volume of 0.4 ml DMEM containing 0.3% BSA for 1 h at 37 °C. The wells were aspirated and washed once with PBS to remove residual virus. Each well was then immediately covered with an agar overlay (final concentration: 1% agar, 1 × MEM, 0.3% BSA and 1 μg ml −1 TPCK-trypsin). The plates were then incubated at 37 °C with 5% CO 2 for 3 days. The overlays were carefully removed and the cells were fixed with 4% paraformaldehyde and permeabilized with 0.5% Triton X-100 for 30 min. The cells were incubated for 1 h with an anti-NP mAb (Abcam) at a 1:1,000 dilution in PBS, followed by a 1-h incubation with peroxidase-conjugated goat anti-mouse IgG (Abcam) at a 1:2,000 dilution and a 30-min incubation with a solution of aminoethylcarbazole (Sigma). Stained plates were scanned and data were recorded. Animal experiments Mice were housed and handled in accordance with the guidelines set by the Association for the Assessment and Accreditation of Laboratory Animal Care. The study protocol was approved by the GIBH Institutional Animal Care and Use Committee. Six-week-old female BALB/c mice were first anaesthetized with isoflurane, and were then inoculated intranasally with 50 μl of virus diluted in PBS. Mock mice were inoculated with 50 μl PBS as control. To test the pathogenicity of IAV-Luc in mice, body weight and survival of mice were monitored daily for 10 days after infection. Mice were humanely killed if the weight loss exceeded 30%. LD 50 values were calculated by Reed–Muench method [19] . Bioluminescence of mice were analysed using Xenogen IVIS200 imaging system (Xenogen Corp.) at the indicated time points. Bioluminescence imaging analysis For imaging of live animals, a stock solution of natural coelenterazine (Promega) was prepared by dissolving the substrate in ethanol to a final concentration of 10 mg ml −1 . At the indicated time points, infected mice were anaesthetized with isoflurane and imaged immediately after tail vein injection at 10 mg/kg of body weight. During imaging, anaesthesia was maintained by nose delivery of isoflurane. Images were acquired with the Xenogen IVIS200 and analysed with the LivingImage 2.11 software package (Xenogen Corp.). For imaging of the lungs, trachea and lung were excised from the euthanized mice at 48 h post infection. A syringe needle was inserted into the opening of the trachea and 0.5 ml of coelenterazine (50 μg ml −1 ) was injected into the lung. After surgical ligation of the trachea, the lungs were imaged using IVIS200. For imaging of viral plaque or cells, confluent MDCK cell monolayers in six-well plates were infected with IAV-Luc or PR8 virus. At 4 days post infection, 1 ml per well of coelenterazine (6 μg ml −1 ) was injected to the underneath of the agar overlay by a 1-ml syringe. The cell culture plates were imaged using IVIS200. Quantification of bioluminescence photon flux The bioluminescence images were analysed with the LivingImage 2.11 software package (Xenogen Corp.). Bioluminescence from samples was quantified by regions of interest (ROI). For mouse imaging, ROIs were drawn by circling regions around the nasopharyngeal turbinate and chest. For cell culture plates, ROIs were drawn by use of standard grids with matrices consistent with multiwell cell culture plates. Signal intensities from ROIs were defined manually and data were expressed as photon flux (photons s −1 cm −2 per sr). Data were presented as mean values±s.e.m. Passive protection of virus-infected mice Antiviral serum was collected from BALB/c mice previous infected with PR8-based virus. Serum was analysed with haemagglutination inhibition (HI) assay. HI assays of sera were performed using chicken erythrocytes by standard method. Sera with HI titre of ≥1280 were pooled and used for passive protection experiments. Female BALB/c mice (three mice per group), 6–8 weeks old, were infected with 50 μl of 10 6 p.f.u. IAV-Luc virus by intranasal inoculation. One hundred microlitres of convalescent sera were injected intravenously via tail vein at 1 h after intranasal challenge. Forty-eight hours after infection, mice were subjected to bioluminescence imaging analysis. Histopathology and immunohistochemistry Lungs from infected and mock mice were collected 5 days post infection and placed into 10% buffered formalin and then embedded in paraffin wax. Six-μm-thick sections were mounted on the slides. Lung sections were stained with haematoxylin and eosin and examined for histopathological changes. For immunohistochemical examination, the sections were stained using an anti-influenza NP mAb (Southern Biotechnology) at a 1:500 dilution, followed by goat anti-mouse IgG, H- and L-chain-specific biotin conjugates (Calbiochem) at a 1:2000 dilution and streptavidin/peroxidase complex reagent (Vector Laboratories). Statistical analysis Statistical significance was determined using unpaired Student’s t -test with two-tailed analysis and the GraphPad Prism 5 software package (GraphPad Software). Data are considered significant when P values are <0.05. How to cite this article: Pan, W. et al. Visualizing influenza virus infection in living mice. Nat. Commun. 4:2369 doi: 10.1038/ncomms3369 (2013).